Performance enhancement of fullerene-based solar cells by light processing A key challenge to the commercialization of organic bulk heterojunction solar cells is the achievement of morphological stability, particularly under thermal stress conditions. Here we show that a low-level light exposure processing step during fabrication of blend polymer:PC 60 BM solar cells can result in a 10-fold increase in device thermal stability and, under certain conditions, enhanced device performance. The enhanced stability is linked to the light-induced oligomerization of PC 60 BM that effectively hinders their diffusion and crystallization in the blend. We thus suggest that light processing may be a promising, general and cost-effective strategy to optimize fullerene-based solar cell performance. The low level of light exposure required suggests not only that this may be an easily implementable strategy to enhance performance, but also that light-induced PC 60 BM oligomerization may have inadvertently influenced previous studies of organic solar cell device behaviour. Recent advances in materials and device design have led to power conversion efficiencies exceeding 9% for solution-processed organic solar cells (OSCs) [1] , approaching the benchmark required for commercial viability. However, increasing the lifetime of plastic photovoltaics remains a major challenge for their commercialization, with both light and heat shown to be stress factors that can induce device degradation [2] . Solution-processed OSCs are typically based on bulk heterojunction films of semiconducting polymers blended with the soluble fullerene derivative PC 60 BM ([6,6]-phenyl-C 61 -butyric acid methyl ester) [3] or its larger analogue PC 70 BM [1] , [4] . The processing, nanomorphology and functional analyses of such films are generally described in terms of the thermodynamics and non-equilibrium assembly of a long-chain macromolecular donor (the polymer) with a small molecule acceptor (the fullerene). A key consideration for the processing and morphological stability of such bulk heterojunction films is therefore the potential of PCBM, as a soluble small molecule, to diffuse through and intercalate within the donor polymer domains [5] , [6] . The high electron affinity and electron mobility of fullerenes have established them as attractive electron acceptors and transport materials for organic electronic devices. Furthermore, their optical absorption in the blue/green region of the solar spectrum, particularly for C 70 derivatives, can contribute significantly to solar light harvesting. Although pristine fullerenes are relatively insoluble, and therefore only amenable to thermal evaporation, derivatized fullerenes such as PCBM can be highly soluble, allowing solution processing and considerable polymer compatibility and miscibility. This contrasts with polymeric acceptors, which typically undergo larger-scale phase segregation when blended with donor polymers, and consequently yield relatively poor solar cell efficiencies [7] . In blend films, fullerenes show a strong tendency to form percolated networks for electron transport, often associated with their three-dimensional symmetry. As a consequence of these advantages, fullerenes are employed almost ubiquitously as the electron acceptor in OSCs. The performance of polymer–fullerene OSCs is strongly dependent on film morphology [8] , [9] , [10] , which is often described as a bicontinuous interpenetrating network of polymer- and fullerene-rich phases. However, numerous studies have emphasized the potential importance of intimately mixed polymer–fullerene domains [11] , [12] , [13] , variations in material crystallinity [14] , [15] and in particular, the presence of relatively pure PCBM domains, and their links to efficient device performance [15] , [16] . More detrimentally, the ability of PCBM molecules, which exhibit weak intermolecular interactions, to diffuse through the blend film is often regarded as the primary cause of thermally induced degradation of solar cell performance [5] , [6] . Under thermal annealing, PCBM molecules have been shown to diffuse within the blend to form micron-sized fullerene crystals [5] , [17] , resulting in severe degradation of device performance. It has been previously established that pristine fullerenes, such as C 60 and C 70 [18] , [19] , and derivatives, such as PCBM [20] , [21] , can undergo photochemical transformation when exposed to visible and, in particular, ultraviolet radiation. Fullerene monomers can be transformed into dimers or higher oligomers, forming covalent intermolecular C–C bonds between fullerene monomers via a ‘2+2 cycloaddition’ mechanism [19] . We have recently reported that C 60 fullerenes are also susceptible to undergo photochemical transformation when blended within inert polymer matrices (polystyrenes, acrylates and so on) [22] . Their photoactive nature, even upon modest ultraviolet or visible irradiation, is effective in suppressing film dewetting, and capable of tuning fullerene nucleation length scales during thermal annealing [22] . Neutron reflectivity indicates that the spatial distribution of fullerenes remains unchanged by light exposure [22] . Light processing of polymer–fullerene composites appears, therefore, as a promising route for the directed assembly of functional materials. With these ideas in mind, we were interested in evaluating the potential impact of fullerene photoinduced oligomerisation on the design and performance of organic solar cells. Employing a benchmark polymer/PC 60 BM blend in films and devices, we demonstrate herein that even modest light exposure (illumination considerably below typical operation conditions) is sufficient to drive a photo-oligomerisation of the PC 60 BM within the blend film which profoundly changes its morphological behaviour, thereby providing both a route to enhance OSC device performance and challenging the relevance of many previous studies of OPV morphological stability (typically conducted in the dark) to practical device operating conditions. Experimental approach We selected a blend of PC 60 BM and benchmark carbazole donor polymer PCDTBT (see Fig. 1a and b for molecular structures) as a model system, and investigated both supported films and functional solar cells. PC 60 BM instead of PC 70 BM was used in blends with PCDTBT, owing to its lower fabrication cost and thus higher commercialization potential, as well as its great tendency for photo-induced crosslinking (at least for C 60 relative to C 70 ) [23] . Devices were fabricated in a conventional architecture without oxide interlayers, thereby avoiding the conductivity effects previously reported following light soaking of devices employing for example ZnO electron collection layers [24] . All light exposure treatments employed a standard low-intensity fluorescent lamp with illumination intensity of ~10 mW cm −2 under nitrogen atmosphere except where specifically stated (see Supplementary Fig. S1 for lamp spectrum). Following irradiation, films and devices were then subjected to thermal stress so as to evaluate the impact of pre-illumination upon the morphological behaviour of the samples. Additional morphological and device studies were carried out with P3HT:PC60BM and DPP-TT-T:PC60BM blends (see Supplementary Fig. S2 and S8 ). 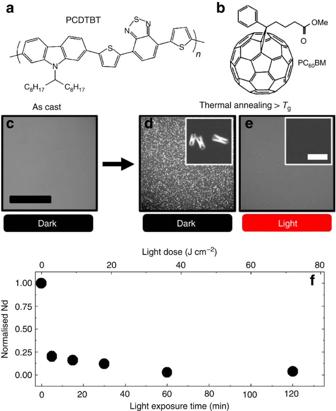Figure 1: Light-induced morphological stabilization. Chemical structures of (a) PCDTBT and (b) PC60BM. Optical microscopy images of PCDTBT:PC60BM (1:2) (c) as-cast blend films (thickness ~80 nm) on silicon substrates (scale bar, 500 μm); (d) after thermal annealing at 140 °C for 1 h (dark) and (e) after thermal annealing at 140 °C for 1 h following fluorescent light treatment (10 mW cm−2, 165 min in N2). The insets (scale bar, 10 μm) to (d) and (e) highlight the drastic difference in the morphologies of annealed blend films without and with light exposure. (f) Shows the number density analysis of PC60BM crystals formed as a function of light dosage following thermal annealing at 140 °C for 1 h. Figure 1: Light-induced morphological stabilization. Chemical structures of ( a ) PCDTBT and ( b ) PC 60 BM. Optical microscopy images of PCDTBT:PC 60 BM (1:2) ( c ) as-cast blend films (thickness ~80 nm) on silicon substrates (scale bar, 500 μm); ( d ) after thermal annealing at 140 °C for 1 h (dark) and ( e ) after thermal annealing at 140 °C for 1 h following fluorescent light treatment (10 mW cm −2 , 165 min in N 2 ). The insets (scale bar, 10 μm) to ( d ) and ( e ) highlight the drastic difference in the morphologies of annealed blend films without and with light exposure. ( f ) Shows the number density analysis of PC 60 BM crystals formed as a function of light dosage following thermal annealing at 140 °C for 1 h. Full size image Light-induced morphological stabilization We begin our study by investigating the effect of light exposure on the morphological behaviour of PCDTBT-PC 60 BM (1:2) blend films under thermal annealing, in conditions analogous and exceeding solar cell operation temperatures. Previous studies have shown that thermal annealing of polymer–fullerene blend films above a threshold temperature results in PC 60 BM diffusion to form micron-sized crystals visible in optical microscopy [6] , [25] . This large-scale crystallization is very detrimental to the device operation, which typically requires nm-sized phase separation [25] . The evolution of film morphology upon annealing above the polymer’s glass transition temperature T g (~106 ° C for PCDTBT), with and without light processing, is shown in Fig. 1 . As-cast blend films are uniform and free of macroscopic PC 60 BM crystallites ( Fig. 1c ). Upon light exposure (in N 2 atmosphere), no morphological changes are observed (data not shown). Upon thermal annealing (140 °C for 1 h in the dark), however, the unexposed ‘dark’ blend film undergoes rapid nucleation and growth of large PC 60 BM crystallites, as shown in Fig. 1d . In particular, ‘chromosome’ shaped PC 60 BM crystallites were formed after this thermal treatment, with a number density of approximately 3500, mm −2 and an average size of 7.5 μm. Remarkably, the number density of such macroscopic crystallites drops drastically in light-treated films upon thermal annealing ( Fig. 1e ). We further note that the temperature of the samples under lamp exposure is less than 35 °C (as measured by surface thermocouple, see Methods section), indicating that the morphological stability is not caused by heating effects during light exposure. It is thus apparent that modest light exposure of PCDTBT:PC 60 BM blend films has had a profound effect on the morphological stability of the film under thermal annealing. The suppression of PC 60 BM crystal formation following light exposure was also observed for other polymer-C 60 and polymer-PC 60 BM systems, including polystyrene:PC 60 BM, P3HT:PC 60 BM and DPP-TT-T:PC 60 BM blends (see Supplementary Fig. S2 ). The suppression was observed for all thermal annealing conditions that gave rise to large-scale PC 60 BM crystallization, including a range of blend compositions, thermal annealing temperatures, substrates and ambient environments (nitrogen and air) (see Supplementary Fig. S3 for selected data). In all cases, low-level light exposure, for periods ranging from a few minutes to a couple of hours, was sufficient to significantly improve morphological stability of the blend films. To quantify the light dose required, we varied the light exposure times and found that 5 min of light exposure could be sufficient to suppress 80% of the PC 60 BM macroscopic crystallization upon thermal annealing, see Fig. 1f . Similarly, exposure to ambient room lights (~0.8 mW cm −2 ) for 16 h in nitrogen was sufficient to suppress 80% of macroscopic crystallites, with this effect being accelerated in the presence of oxygen (see Supplementary Fig. S3 for selected data). This high sensitivity to light exposure suggests that the photochemical transformation driving this increase in morphological stability can be remarkably efficient. It is thus apparent that even modest inadvertent exposure to ambient lighting may have a significant impact on the morphological stability of polymer:PCBM blend films during device processing and subsequent storage/operation. Direct evidence of PC 60 BM oligomerization Previous studies have suggested that light exposure of C 60 and PC 60 BM films can result in fullerene oligomerization, thereby substantially reducing their solubility [18] , [26] . Such fullerene oligomerization is therefore the most probable origin of the enhanced morphological stability of PCDTBT:PC 60 BM blend films following light exposure reported above. Direct evidence for such PC 60 BM oligomerization under the light exposure conditions employed in Fig. 1 is provided via gel permeation chromatography (GPC) and Raman measurements. GPC experiments were performed to detect the change in the molecular weight of the blend materials and its constituents, as the formation of new chemical bonds between PC 60 BM during light exposure should be reflected by the emergence of a new GPC peak corresponding to PC 60 BM oligomers. Measurements were done by re-dissolving the spin-casted PCDTBT-PC 60 BM (1:2) films following 4 h light exposure in N 2 . As shown in Fig. 2a , no change was observed for the PCDTBT signal (peak i), suggesting that the PCDTBT phase was not involved in the photochemical transformation process. An extra peak (peak iii) at a molecular mass two to three times that of PC 60 BM (peak ii) is observed following light exposure, confirming the formation of PC 60 BM oligomers. 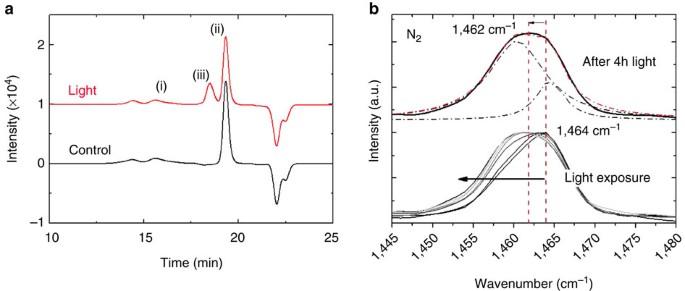Figure 2: Direct evidence of PC60BM oligomerization. (a) Gel permeation chromatography data for the PCDTBT:PC60BM (1:2) blend samples with and without light exposure. Control data for the individual film components (seeSupplementary Fig. S4) allows us to assign these peaks to (i) PCDTBT, (ii) PC60BM and (iii) PC60BM species generated by light exposure. (b) Top: Raman data at 488 nm excitation wavelength (10 s acquisition time) for neat PC60BM film after being exposed to 4 h of fluorescent light. The data is fitted by two Lorentzian functions with peak positions at ~1,460 cm−1(oligomerized PC60BM) and ~1,465 cm−1(pristine PC60BM), respectively. Bottom: sequentially collected Raman spectra for initially dark PC60BM film under continuous 488 nm laser exposure for 10, 30, 50, 70 and 110 s. Figure 2: Direct evidence of PC 60 BM oligomerization. ( a ) Gel permeation chromatography data for the PCDTBT:PC 60 BM (1:2) blend samples with and without light exposure. Control data for the individual film components (see Supplementary Fig. S4 ) allows us to assign these peaks to (i) PCDTBT, (ii) PC 60 BM and (iii) PC 60 BM species generated by light exposure. ( b ) Top: Raman data at 488 nm excitation wavelength (10 s acquisition time) for neat PC 60 BM film after being exposed to 4 h of fluorescent light. The data is fitted by two Lorentzian functions with peak positions at ~1,460 cm −1 (oligomerized PC 60 BM) and ~1,465 cm −1 (pristine PC 60 BM), respectively. Bottom: sequentially collected Raman spectra for initially dark PC 60 BM film under continuous 488 nm laser exposure for 10, 30, 50, 70 and 110 s. Full size image Figure 2b shows the Raman spectra of pristine PC 60 BM and photo-oligomerized PC 60 BM films. The peak position of the Ag (2) Raman mode can be used to distinguish pristine PC 60 BM and PC 60 BM oligomers, with characteristic peak positions at 1,465 and 1,460 cm −1 respectively [27] . Peak analysis of the Raman signal for pristine and fluorescent light-exposed PC 60 BM film indicates an increased fraction of PC 60 BM oligomers in the latter sample (see top curve in Fig. 2b ). For the pristine sample we observed a gradual shift in the peak positions of the PC 60 BM Ag (2) mode from 1,464 to 1,461 cm −1 following exposure to the 488-nm excitation laser (exposure time 10–110 s) indicating that the PC 60 BM are photo-oligomerized in situ by the 488-nm laser (see Fig. 2b bottom curve). The PCBM oligomerization reported above does not appear to have a significant impact upon its photophysical properties. Light exposure of neat PC 60 BM films under inert atmosphere, analogous to that employed in Figs 1 and 2 , was observed to have no measurable impact on the PCBM optical absorption, and only a small redshift (~5 nm) of the emission properties (see Supplementary Fig. S5 ). It thus appears that light-induced PC 60 BM oligomerization does not substantially affect its electronic properties, at least in terms of its highest occupied (HOMO) and lowest unoccupied molecular orbital (LUMO) energies. Device performance enhancement by light processing We now consider the impact of light-induced PC 60 BM oligomerization on the performance of benchmark PCDTBT:PC 60 BM OSCs. We address two issues: first the impact of this oligomerization process upon the stability of these devices under modest thermal stress; and second the potential of this oligomerization as a processing step to enhance the performance of suboptimal OSC devices. Several studies have reported that PCBM diffusion is a key factor related to the stability of OSC devices under thermal stress [2] , [5] , [6] . Although for P3HT:PC 60 BM-based organic photovoltaic devices, it has been shown that limited thermal annealing can enhance performance, for devices based on most higher efficiency donor polymers, such as PCDTBT employed herein, thermal annealing typically results in degradation of the device performance. Our stability studies employed an 80°C dark thermal stress. Devices were fabricated in a standard architecture on ITO/PEDOT:PSS substrates, with a light exposure step (>120 min) introduced either before or after evaporation of a Ca/Al top electrode. The stability of completed cells was measured using repeated dark thermal annealing/room temperature device measurement cycles. For the current–voltage ( J–V ) measurements, the devices were exposed under a solar simulator for less than 30 s to minimize the effect of PC 60 BM oligomerization caused by this simulated solar irradiation. The samples were otherwise kept under dark conditions to eliminate any variations in experimental conditions. 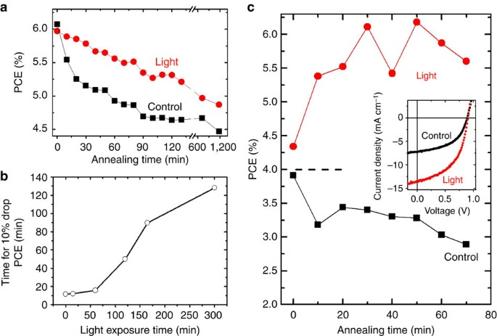Figure 3: Device performance enhancement by light processing. Analyses of PCDTBT:PC60BM solar cell PCE as a function of thermal annealing and light exposure times. PCE data in (a) and (c) are shown as a function of annealing time at 80 °C following a fixed light exposure (2.75 h of white light 10 mW cm−2) as well as control data without light exposure. Plot (a) shows data for devices fabricated with optimized film deposition, whereas (c) shows data for devices with non-optimized spin-coating conditions (and therefore lower initial efficiencies). The inset to plot (c) compares theJ–Vcharacteristics of the non-optimized devices in (c) with and without light exposure followed by thermal annealing at 80 °C for 50 min. Plot (b) shows the annealing time required for a 10% PCE loss of initially optimized devices as a function of light exposure time. Further details of device performance characteristics and data reproducibility are given inSupplementary Fig. S6. Figure 3a addresses the impact of light treatment on the initial 80 °C thermal stability of a pair of typical optimized PCDTBT:PC 60 BM devices (see Supplementary Fig. S6 for data averaged over five sample batches). Light treatment alone, in the absence of any heat treatment, was observed to have negligible impact on device efficiency. For the devices fabricated without light treatment, a rapid decrease in device performance was observed, with their power conversion efficiency (PCE) dropping by 10% after only 11 min of 80 °C thermal annealing. This drop in PCE was primarily caused by a rapid drop in device fill factor (FF), accompanied by drops in both short circuit current ( J sc ) and open circuit voltage ( V oc ) (see Supplementary Fig. S6 ), in agreement with previous stability studies [28] . In contrast, devices fabricated with light treatment exhibited significantly enhanced stability, taking ~120 min for the PCE to drop by 10%. The enhanced device stability is due to a much slower decrease in FF, accompanied by a small increase in V oc during the thermal stress process. This photo-induced stability enhancement was also observed in longer timescale trials employing 20 h of thermal stress (see Fig. 3a ). To quantify the effect of light dose on device thermal stability, we varied the light exposure time and observed a steady increase in device lifetime with increasing controlled light exposure time; see Fig. 3b . It is apparent that a somewhat longer light exposure time is required to enhance device stability compared with that required to inhibit macroscopic PC 60 BM crystallization in films annealed above T g ( Fig. 1d ). Nevertheless, only 150 min of 10 mW cm −2 white light irradiation was sufficient to substantially enhance device morphological stability. Similar stability data were also obtained for light treatment before or after electrode deposition (see Supplementary Fig. S7 ). It is thus apparent that the PC 60 BM oligomerization and the associated enhanced morphological stability induced by modest light exposure during device fabrication (as observed in Figs 1 and 2 ) results in an approximately 10-fold increase in the overall stability of these benchmark OSCs under thermal stress conditions. Figure 3: Device performance enhancement by light processing. Analyses of PCDTBT:PC 60 BM solar cell PCE as a function of thermal annealing and light exposure times. PCE data in ( a ) and ( c ) are shown as a function of annealing time at 80 °C following a fixed light exposure (2.75 h of white light 10 mW cm −2 ) as well as control data without light exposure. Plot ( a ) shows data for devices fabricated with optimized film deposition, whereas ( c ) shows data for devices with non-optimized spin-coating conditions (and therefore lower initial efficiencies). The inset to plot ( c ) compares the J–V characteristics of the non-optimized devices in ( c ) with and without light exposure followed by thermal annealing at 80 °C for 50 min. Plot ( b ) shows the annealing time required for a 10% PCE loss of initially optimized devices as a function of light exposure time. Further details of device performance characteristics and data reproducibility are given in Supplementary Fig. S6 . Full size image The observed enhancement in device stability is not specific to PCDTBT:PC 60 BM devices; an analogous enhancement of morphological stability was also observed for devices employing the low-bandgap polymer DPP-TT-T blended with PC 60 BM (see Supplementary Fig. S8 ). These data show that the light-induced enhanced morphological stability apparent from our PC 60 BM crystallization studies above T g in films also extends to enhanced photovoltaic device stability under temperature stress conditions relevant to practical device performance. We finally consider the potential use of light treatment as a processing step to optimize and enhance device performance. Thermal annealing is widely used as a processing step to tune blend morphology and improve performance of as-cast, non-equilibrium films. Thermal annealing has been shown to be an effective processing step for P3HT:PCBM solar cells [29] , but has not been previously shown to be effective in enhancing the efficiency of PCDTBT:PCBM devices. Figure 3c demonstrates the potential impact of light treatment upon such thermal annealing processing for PCDTBT:PC 60 BM devices, employing suboptimal film deposition conditions such that the initial device performance is relatively poor (PCE of~4%, see Methods for experimental details). It is apparent that for a device fabricated without light treatment, thermal annealing resulted in a monotonic decrease in device performance with increasing annealing time (and annealing temperature, data not shown), consistent with previous studies [28] , and with Fig. 3c . In contrast, the device fabricated with a light treatment shows a 44% increase in device performance with PCE increasing from 4.3 to 6.2% following thermal annealing at 80 ° C for 1 h, followed by a drop in PCE with further annealing. The increase in PCE is primarily due to an increase in short circuit current ( J sc ), accompanied by a mild increase in both V oc and FF (see Supplementary Fig. S9 ). This drastic increase in PCE for the device with light treatment is noteworthy, and has not been observed before for PCDTBT:PCBM blends. This increase is most probably caused by the oligomerization of PC 60 BM preventing the diffusion of PC 60 BM, whereas thermal annealing enhances the ordering of the polymer phase [30] . A more optimized blend morphology is also consistent with an increased J sc and FF due to better charge generation and collection. Thermally induced morphological degradation is a key consideration for commercial application of organic bulk heterojunction solar cells. In this paper, we have reported that modest light irradiation of a benchmark polymer–fullerene blend can result in substantially enhanced morphological stability under subsequent thermal stress for both films and complete solar cells. Evidence is presented linking this enhanced stability with photo-induced PC 60 BM oligomerization. The magnitude of the stabilization is observed to depend on the details of film composition, annealing temperature, substrate and so on. Nevertheless, it is striking that under the conditions studied only a few minutes of modest irradiation (~1/10th of standard solar irradiation intensity) was sufficient to suppress almost completely thermally induced PC 60 BM macroscopic crystallization in a benchmark polymer: PC 60 BM film, and that 100 min of such modest irradiation was sufficient to increase device longevity under subsequent thermal stress by an order of magnitude. It should be noted that recent studies on the stability of polymer–fullerene solar cells under thermal stress have reported substantial variations in performance (with, for example, times for 10% loss of PCE under thermal stress ranging from tens of minutes to ≳ 100 h (refs 31 , 32 , 33 , 34 )). The origins of these variations are not fully resolved, but most probably related to details of device fabrication (for example, photoactive layer and electrode composition) and experimental measurement conditions (for example, light exposure, temperature, pre-evaluation initial device annealing). For example, our own studies have indicated that the longer lifetimes reported in Bertho et al. [32] are most probably related to the use a pre-evaluation annealing step, so excluding any initial performance degradation from their study, and due to the use of PC 70 BM as an electron acceptor (which is reported to have superior morphological stability in blend films than PC 60 BM [35] , [36] ). The stability data we report herein is clearly limited in scope and timescale, but unequivocally demonstrates that light exposure can have a positive impact upon thermal stability. For long-term stability enhancement, it is likely that continuous irradiation during thermal stress will be necessary to maintain PCBM oligomerization (prolonged thermal annealing has been shown to reverse photo-induced C 60 cross-linking [18] ). Such combined light and thermal stress is of particular relevance to practical solar cell operating conditions (continuous irradiation is likely to be particularly important for devices employing PC 70 BM as previous studies have indicated C 70 is less susceptible to photo-induced crosslinking than C 60 (ref. 23 ). Indeed it appears possible that the impressive device lifetimes reported for analogous PCDTBT:PCBM devices under solar irradiation (projected lifetimes of ~6 years [37] ) may in part be related to photo-induced PCBM oligomerization ensuring a stable film morphology. The main conclusions of the paper are summarized graphically in Fig. 4 ; an additional ‘light annealing’ step during fullerene-based OSC fabrication can significantly improve device lifetime and optimize performance. The light exposure causes oligomerization of PC 60 BM, which then imparts greater film morphological stability under subsequent heat stress or thermal annealing. This effect is robust to all polymer matrices and temperatures studied. We show that even modest illumination, commensurate with typical laboratory conditions, is sufficient to initiate this effect and must therefore be monitored and controlled to ensure consistent device performance. As such, inadvertent light exposure is likely to have significantly impacted many previous studies of OSC morphological behaviour employing acceptor fullerenes. Several studies have reported the synthesis of new active layer materials that enable photo-induced polymerization or crosslinking approaches to enhance OSC device stability [38] , [39] . However, these approaches typically require increases in materials complexity and/or a loss of device efficiency. The findings reported herein suggest that photo-induced oligimerization may be readily achieved with materials already employed in optimized devices, with negligible loss of performance, thereby providing an attractive route to enhancing the commercial potential of OSCs. 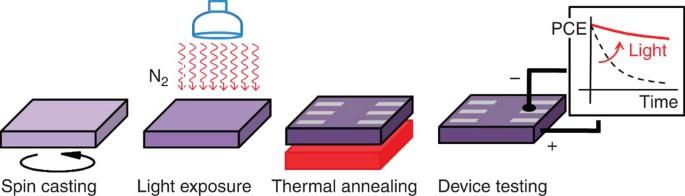Figure 4: Proposed experimental procedure for OSC device fabrication and stability studies. An additional controlled low-level ‘light annealing’ step in OSC device fabrication results in significantly enhanced device thermal stability and/or enhanced device performance. Figure 4: Proposed experimental procedure for OSC device fabrication and stability studies. An additional controlled low-level ‘light annealing’ step in OSC device fabrication results in significantly enhanced device thermal stability and/or enhanced device performance. Full size image Materials PCDTBT was supplied by 1-materials and purified at Imperial with a molecular weight ( M w ) of 21.6 kg mol −1 and polydispersity of 5.5. PC 60 BM was supplied by Nano-C. The midpoint T g of neat PCDTBT was measured as 106±1 °C using differential scanning calorimetry (DSC TA Instruments Q2000) at the rate of 10 °C min −1 . Morphological stability studies Silicon substrates (Compart Technology) were cleaned with N 2 before use. Samples were made by spin-casting the active bulk heterojunction layer comprising weight ratio 1:2 PCDTBT:PC 60 BM on to silicon substrates with a thickness of 80 nm. A fluorescent lamp was used as the light source, with light intensity and spectrum measured by a StellarNet EPP2000 spectrometer. Blend film morphology was observed by a reflection optical microscope (Olympus BX 41M), equipped with an XY stage and CCD camera (AVT Marlin). Gel permeation chromatography GPC measurements were performed using Agilent Technologies 1,200 series GPC running in chlorobenzene at 80 °C, using two PL mixed B columns in series, and calibrated against narrow polydispersity polystyrene standards. Raman spectroscopy Raman measurements were performed using a Renishaw In-Via Raman microscope in a back-scattering configuration on PC 60 BM neat and blend samples; the latter spectra are dominated by the polymer signal, which does not change upon illumination. The excitation wavelength is 488 nm with a power of ~0.9 mW and a beam diameter of ~10 μm on the films. All the measurements were done in nitrogen environment to reduce the competing fullerene photo-oxidation process. In all cases, the spectra were obtained with data acquisition time of 10 s, unless specified. The Raman spectra were background corrected using the Renishaw Wire 3.1 program. The spectral resolution is ~1 cm −1 . Device fabrication and stability study ITO glass substrates were cleaned by sonication in deionized water, acetone and isopropyl alcohol (IPA) successively, followed by an oxygen plasma treatment at 100 W for 7 min before a 35-nm-thick PEDOT:PSS layer was deposited on to the substrates and then annealed at 150 °C for 20 min. The substrates were then transferred to N 2 glovebox for deposition of the active layer. A number of device fabrication recipes were employed varying the dissolving solvent, weight ratio, solution concentration, dissolving period, spin acceleration and spin speed. For the PCDTBT:PC 60 BM devices fabricated in Fig. 3a , PCDTBT and PC 60 BM were codissolved in anhydrous chlorobenzene with a total solution concentration of 25 mg ml −1 and a weight ratio of 1:2. For the PCDTBT:PC 60 BM devices fabricated in Fig. 3c , PCDTBT and PC 60 BM were codissolved in anhydrous dichlorobenzene with a total solution concentration of 40 mg ml −1 and a weight ratio of 1:2. Solutions were stirred in N 2 glovebox at 55 °C for more than 24 h followed by filtering through a 0.2-μm filter. Active layer film thickness is ~85-nm thick for the devices fabricated in Fig. 3a and ~80-nm thick for the devices fabricated in Fig. 3c . All devices were completed by evaporation of 25 nm of calcium and 100 nm of aluminium through a 6-pixel mask. The pixel size, defined by the spatial overlap of the ITO anode and Ca/Al cathode, was 0.045 cm 2 . Film thickness was determined with a Dektak 6M profilometer. Annealing steps in both morphology and device stability studies were carried out in a N 2 -filled glovebox. For device degradation studies, the same lamp was used for light exposure as the morphological studies. Annealing temperature was measured and calibrated using a Kane–May KM330 temperature sensor. The film surface temperature under illumination was measured with a surface thermocouple connected to the films on silicon or ITO/PEDOT:PSS substrates. J–V characteristics were measured using a Xenon lamp at AM1.5 solar illumination (Oriel Instruments) calibrated to a silicon reference cell with a Keithley 2,400 source meter. How to cite this article: Li, Z. et al. Performance enhancement of fullerene-based solar cells by light processing. Nat. Commun. 4:2227 doi: 10.1038/ncomms3227 (2013).